ANKS6 is the critical activator of NEK8 kinase in embryonicsitusdetermination and organ patterning The ciliary kinase NEK8 plays a critical role in situs determination and cystic kidney disease, yet its exact function remains unknown. In this study, we identify ANKS6 as a target and activator of NEK8. ANKS6 requires NEK8 for localizing to the ciliary inversin compartment (IC) and activates NEK8 by binding to its kinase domain. Here we demonstrate the functional importance of this interaction through the analysis of two novel mouse mutations, Anks6 Streaker and Nek8 Roc . Both display heterotaxy, cardiopulmonary malformations and cystic kidneys, a syndrome also characteristic of mutations in Invs and Nphp3 , the other known components of the IC. The Anks6 Strkr mutation decreases ANKS6 interaction with NEK8, precluding NEK8 activation. The Nek8 Roc mutation inactivates NEK8 kinase function while preserving ANKS6 localization to the IC. Together, these data reveal the crucial role of NEK8 kinase activation within the IC, promoting proper left–right patterning, cardiopulmonary development and renal morphogenesis. Physiologic ciliary architecture and function is contingent on the proper interaction of specific multimeric protein complexes, which regulate cilium-specific biochemical processes [1] , [2] , [3] , [4] . Although modules such as the NPHP1-4-8 complex, the MKS complex, IFT particles and the BBSome fulfill gatekeeping and protein transport functions, the biological role of the ciliary inversin compartment (IC) remains unknown. Although the known IC proteins inversin (INVS), NPHP3, NEK8 and ankyrin repeat and SAM domain-containing protein 6 (ANKS6) are unnecessary for ciliogenesis, nonsense mutations or genetic knockouts result in severe multiorgan malformation syndromes, embryonic or perinatal lethality, left–right asymmetry perturbations, cardiopulmonary defects and cystic kidneys [5] , [6] , [7] , [8] , [9] . Missense mutations in IC genes are also associated with cystic kidney disease [10] , [11] , [12] , [13] , [14] , [15] . The IC protein NEK8 stands out as the only ciliary axonemal kinase and was characterized as a cystic kidney disease protein in rodents and humans [10] , [14] , [16] . Similar to other IC genes, mice with a Nek8 deletion exhibit a syndrome of perinatal lethality, cardiac defects, renal glomerulocystic disease and left–right asymmetry randomization [6] . Although a recent study has identified a role for NEK8 kinase function in DNA replication [17] , the mechanism of NEK8-dependent ciliopathy is unknown, nor are there reports of physiologic phosphorylation substrates in cilia. In fact, none of the cystogenic missense mutations of NEK8 reside in its kinase domain. It has therefore remained unclear whether NEK8 kinase activity is necessary for its biologic function in ciliary signalling and development. In the present study, we aimed to characterize NEK8 with respect to its functions as a kinase, identify phosphorylation targets and investigate kinase-specific signalling in the pathogenesis of an IC-specific ciliopathy syndrome. We show that ANKS6 and NEK8 form a highly stable subcomplex within the IC protein interaction network, and that the ANKS6–NEK8 interaction results in phosphorylation of ANKS6 and in a strong stimulation of NEK8 kinase activity. We present two novel mouse missense mutations in Nek8 and Anks6 , respectively, that independently give rise to a severe heterotaxy syndrome with cardiopulmonary malformations and polycystic kidney disease, phenocopying the full genetic knockout of IC genes. The biochemical consequence of the Anks6 mutation is revealed as a loss in NEK8-binding affinity, leading to reduced kinase activation, while the Nek8 mutation directly inactivates kinase function. Together, our data demonstrate the importance of NEK8 kinase activity and its regulation through ANKS6 in left–right asymmetry determination, and proper cardiopulmonary and renal tissue morphogenesis. ANKS6 stimulates NEK8 phosphorylation activity To identify interaction partners of NEK8, we performed large-scale immunoprecipitation (IP) experiments from mIMCD3 cells stably expressing FLAG-NEK8. On SDS–polyacrylamide gel electrophoresis (SDS–PAGE) and silver staining ( Fig. 1a ), two signals near 75 and 110 kDa were identified by mass spectrometry as NEK8, the bait protein, and the ANKS6, respectively. When we subjected total FLAG-NEK8 and control murine intramedullary collecting duct (IMCD) cell immunoprecipates to direct mass spectrometric analysis, we confirmed ANKS6 as binding partner, along with other proteins ( Fig. 1b ). We focused our attention on ANKS6, the gene product mutated in the Han:SPRD cy/+ rat model of polycystic kidney disease [11] , which was recently found to be an IC protein responsible for a human autosomal-recessive nephronophthisis-like syndrome [18] . As in Hoff et al . 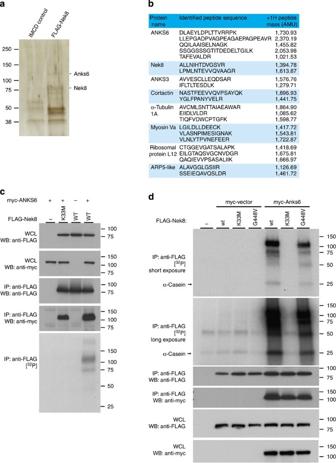Figure 1: ANKS6 interacts with NEK8, enhancing NEK8 kinase activity. (a) IP of FLAG-NEK8 from mIMCD3 cells stably transduced with a retroviral FLAG-NEK8 expression construct reveals a number of distinct co-precipitating bands on silver stain. ANKS6 is identified by mass spectrometry. (b) Mass spectrometric analysis of the FLAG-IP eluate reveals a number of distinct peptide fingerprints, among which ANKS6 was elected as an interesting candidate protein for further analysis. (c) ANKS6 co-precipitates with NEK8, is phosphorylated by NEK8 and promotes NEK8 autophosphorylation in an IP/kinase assay. No phosphorylation activity was observed in the absence of ANKS6, or in the setting of a K33M ‘kinase-dead’ allele. (d) ANKS6 enhances kinase activity of wild-type NEK8, as well as the pathogenic NEK8jckmutant, towards itself, the kinase, and towards α-casein, a nonspecific phosphorylation substrate. [18] , we confirmed that morpholino-induced knockdown of ANKS6 in zebrafish results in laterality defects reminiscent of NEK8 morphant phenotypes [6] ( Supplementary Table 1 ). Figure 1: ANKS6 interacts with NEK8, enhancing NEK8 kinase activity. ( a ) IP of FLAG-NEK8 from mIMCD3 cells stably transduced with a retroviral FLAG-NEK8 expression construct reveals a number of distinct co-precipitating bands on silver stain. ANKS6 is identified by mass spectrometry. ( b ) Mass spectrometric analysis of the FLAG-IP eluate reveals a number of distinct peptide fingerprints, among which ANKS6 was elected as an interesting candidate protein for further analysis. ( c ) ANKS6 co-precipitates with NEK8, is phosphorylated by NEK8 and promotes NEK8 autophosphorylation in an IP/kinase assay. No phosphorylation activity was observed in the absence of ANKS6, or in the setting of a K33M ‘kinase-dead’ allele. ( d ) ANKS6 enhances kinase activity of wild-type NEK8, as well as the pathogenic NEK8 jck mutant, towards itself, the kinase, and towards α-casein, a nonspecific phosphorylation substrate. Full size image As no physiological substrate of NEK8 has been described to date, we asked whether ANKS6 might represent a target for NEK8-mediated phosphorylation. Under our experimental conditions, NEK8 did not exhibit any significant phosphorylation activity after IP from transiently transfected 293T cells. However, co-expression of ANKS6 resulted in a strong autoradiographic signal at ~100 kDa, consistent with ANKS6 phosphorylation, as well as an ~75-kDa signal, consistent with autophosphorylation of NEK8 in the presence of ANKS6. When ANKS6 was coprecipitated with NEK8 K33M , an engineered ‘kinase-dead’ allele of NEK8, neither phosphorylation activity towards ANKS6 nor NEK8 autophosphorylation was observed, while ANKS6 binding was unaffected ( Fig. 1c ; see Supplementary Fig. 1 for details on kinase assay parameters and IP). To our knowledge, this provides the first description of an endogenous ciliary substrate of the NEK8 kinase. As the addition of ANKS6 resulted in increased NEK8 kinase activity against both ANKS6 and NEK8, we asked whether ANKS6 is also capable of stimulating NEK8 kinase activity against other substrates. By using α-casein as a generic kinase substrate, we indeed observed NEK8-dependent incorporation of radioactive phosphate in the presence of ANKS6 ( Fig. 1d ). In the case of the NEK8 G448V (jck) mutant protein, kinase activity appeared similar when compared with the wild type (also Supplementary Fig. 4d , in contrast to Choi et al . [17] ), but remained dependent on ANKS6. Importantly, we did not observe any incorporation of 32 P in either NEK8 or α-casein in the absence of ANKS6. As neither full-length NEK8 nor ANKS6, nor truncation constructs are soluble when expressed in bacteria, we were unable to perform in vitro phosphorylation assays with purified, recombinant proteins. Given that phosphorylation activity is strictly dependent on both the presence of ANKS6 and a functional NEK8 allele (and, as shown below, specific domains of each protein), it is highly unlikely that the kinase activity originates from a co-precipitating contaminant. We therefore postulate that ANKS6 is not only an interaction partner and substrate of NEK8, but also a functional activator of NEK8 kinase activity. NEK8 kinase domain is necessary for interaction with ANKS6 Given the distinct functions of ANKS6 related to NEK8 kinase activity, we investigated the nature of the NEK8/ANKS6 interaction in greater detail. We designed a set of amino- and carboxy-terminal truncations of NEK8, generating partially overlapping fragments of kinase- and RCC1-repeat domain, to be employed in co-IP assays with ANKS6 ( Fig. 2a ). ANKS6 bound to the full-length wild-type NEK8 protein, as well as to truncation variants that include the kinase domain and a short C-terminal extension ( Fig. 2b ), consistent with a functional role of ANKS6 in NEK8 kinase activation. In contrast, interaction of NEK8 with INVS is mediated by the RCC1-repeat domain: a truncation variant that contains all seven predicted RCC1 repeats, as well as a shorter truncation comprising five C-terminal RCC1 repeats both bound to INVS, while the kinase domain did not appear necessary for this interaction ( Fig. 2c ). On closer analysis, the kinase domain alone did not reveal measurable phosphorylation activity, while NEK8 1-295 and NEK8 1-415 , two minimal ANKS6-binding truncation variants, were fully active in the complex with ANKS6 ( Fig. 2d ). Again, phosphorylation of α-casein, ANKS6 and the respective NEK8 truncation mutant occurred only in the presence of ANKS6. 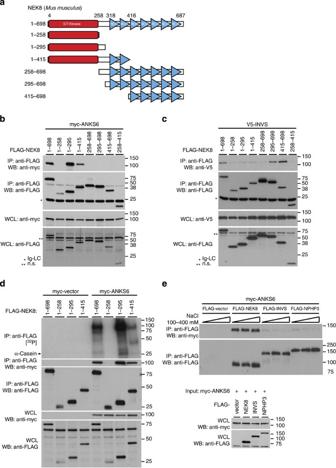Figure 2: ANKS6 exerts its kinase stimulating activity through direct interaction with the NEK8 kinase domain. (a) NEK8 truncations were employed in IP/binding assays, to map interaction sites. (b) The kinase domain of NEK8, along with a short C-terminal extension (NEK81-295) mediates the interaction with ANKS6, while the RCC1 domain does not contribute to complex formation. (c) NEK8 interacts with inversin through its RCC1 domain; the five C-terminal RCC1 repeats (amino acids 416–698), in particular, are necessary and sufficient for binding. (d) The NEK8 kinase domain (NEK81-258), as predicted by homology alignment, is not capable of binding ANKS6 and is inactive as a kinase. NEK81-295, a larger truncation that binds ANKS6, exhibits dramatically enhanced phosphorylation activity. The full-length wild-type NEK8 and the NEK81-415truncation are included as controls. Any phosphorylation is only detected in the presence of ANKS6, generating autoradiographic signals at the levels of ANKS6 (100 kDa), α-casein (25 kDa) and the molecular weight of the respective NEK8 truncations. (e) Co-IP of myc-ANKS6 with FLAG-NEK8, -INVS and -NPHP3, and fractionation with different ionic strength conditions demonstrates formation of a salt-insensitive robust subcomplex between NEK8 and ANKS6. Figure 2: ANKS6 exerts its kinase stimulating activity through direct interaction with the NEK8 kinase domain. ( a ) NEK8 truncations were employed in IP/binding assays, to map interaction sites. ( b ) The kinase domain of NEK8, along with a short C-terminal extension (NEK8 1-295 ) mediates the interaction with ANKS6, while the RCC1 domain does not contribute to complex formation. ( c ) NEK8 interacts with inversin through its RCC1 domain; the five C-terminal RCC1 repeats (amino acids 416–698), in particular, are necessary and sufficient for binding. ( d ) The NEK8 kinase domain (NEK8 1-258 ), as predicted by homology alignment, is not capable of binding ANKS6 and is inactive as a kinase. NEK8 1-295 , a larger truncation that binds ANKS6, exhibits dramatically enhanced phosphorylation activity. The full-length wild-type NEK8 and the NEK8 1-415 truncation are included as controls. Any phosphorylation is only detected in the presence of ANKS6, generating autoradiographic signals at the levels of ANKS6 (100 kDa), α-casein (25 kDa) and the molecular weight of the respective NEK8 truncations. ( e ) Co-IP of myc-ANKS6 with FLAG-NEK8, -INVS and -NPHP3, and fractionation with different ionic strength conditions demonstrates formation of a salt-insensitive robust subcomplex between NEK8 and ANKS6. Full size image To further define the relationship of IC components, we tested binary protein–protein interactions between ANKS6 and NEK8, INVS and NPHP3 in co-IP assays, and challenged immunocomplexes with different ionic strengths. ANKS6 bound to both INVS and NPHP3 under low stringency conditions; however, these interactions were easily dissociated by raising the ionic strength to an equivalent of 250 mM NaCl or above ( Fig. 2e ). In contrast, the interaction of ANKS6 with NEK8 demonstrated extraordinary stability, withstanding cell lysis and co-precipitation at 400 mM NaCl without any decrease in binding. Although the assay conditions are above physiologic concentrations of intracellular ions, the results indicate that NEK8 and ANKS6 constitute a distinct subcomplex within the IC interaction network. We also performed kinase assays with NEK8 and combinations of INVS, NPHP3 and ANKS6, to test whether INVS or NPHP3 serve as substrates or modulators of NEK8 kinase activity ( Supplementary Fig. 2 ). INVS and NPHP3 alone or in combination did not alter NEK8 activity, nor did they appear to serve as phosphorylation substrates, even when ANKS6 was present. ANK-repeat domain of ANKS6 is necessary for NEK8 activation The ANKS6 protein spans 885 amino acids, involving an N-terminal domain of ten ankyrin repeats (ANK), as well as a C-terminal sterile α-motif (SAM), separated by an ~300 amino acid region without any identifiable structural features ( Fig. 3a ). We found the ANK-repeat domain of ANKS6 to be necessary for interaction with NEK8 ( Fig. 3b ), while truncation of the SAM domain or larger C-terminal portions of ANKS6 did not affect NEK8 binding. All ANKS6 truncations capable of NEK8 binding were also readily phosphorylated. Aiming to map the interaction region more precisely, we selectively introduced truncations along ANK-repeat boundaries within the ANK-repeat domain. NEK8 binding was lost when the four N-terminal ANK repeats were deleted, while truncation of only the first N-terminal ANK repeat resulted in only a minor reduction of NEK8 binding ( Fig. 3c ). 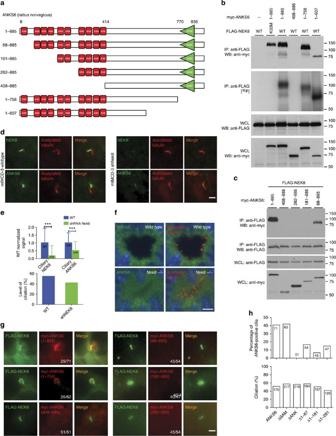Figure 3: The ankyrin-repeat domain of ANKS6 is necessary for NEK8 binding and targeting of ANKS6 to the IC. (a) Different ANKS6 truncations were employed in IP/binding assays and IF. (b) ANKS6 interacts with NEK8 through its ANK-repeat domain, while the SAM domain is not essential for binding. ANKS6 truncations that interact with NEK8 are readily phosphorylated in complex with NEK8. (c) A truncation variant of ANKS6 lacking the first ANK repeat binds to NEK8, while truncation of the first four ANK repeats completely abrogates binding. (d,e) Short hairpin RNA (shRNA)-mediated targeted knockdown of NEK8 significantly reduces the ciliary ANKS6 signal. IF signal intensities were compared between wild-type IMCD cells and IMCDshNek8cells, for both anti-NEK8 and anti-ANKS6 signals (scale bar, 2 μm). The number of individual cilia analysed is indicated in the respective bar. Differences were highly significant by Student’st-test, withP<0.01 (upper bar graph). The total level of ciliation is only mildly affected by Nek8 knockdown (lower bar graph; percentage of numeric counts of ciliated cells over total cells). (f) Fluorescence immunohistochemistry on kidney sections of wild-type (upper panels) andNek8−/−mice (lower panels), employing antibodies against ANKS6 (green) and acetylated tubulin (red). Positive ANKS6 signals at the ciliary base can only be identified in the wild type, not inNek8−/−cilia (scale bar, 5 μm). (g,h) Coexpression of myc-tagged ANKS6 truncation variants and FLAG-tagged wild-type NEK8 demonstrates the importance of the ANK-repeat domain for NEK8 binding and consecutive ciliary targeting of ANKS6 (scale bar, 2 μm; upper bar graph, percentage of numeric counts of ANKS6-positive cilia over total cilia; lower bar graph, percentual level of ciliation; the number of cells counted is indicated in each bar). Figure 3: The ankyrin-repeat domain of ANKS6 is necessary for NEK8 binding and targeting of ANKS6 to the IC. ( a ) Different ANKS6 truncations were employed in IP/binding assays and IF. ( b ) ANKS6 interacts with NEK8 through its ANK-repeat domain, while the SAM domain is not essential for binding. ANKS6 truncations that interact with NEK8 are readily phosphorylated in complex with NEK8. ( c ) A truncation variant of ANKS6 lacking the first ANK repeat binds to NEK8, while truncation of the first four ANK repeats completely abrogates binding. ( d , e ) Short hairpin RNA (shRNA)-mediated targeted knockdown of NEK8 significantly reduces the ciliary ANKS6 signal. IF signal intensities were compared between wild-type IMCD cells and IMCD shNek8 cells, for both anti-NEK8 and anti-ANKS6 signals (scale bar, 2 μm). The number of individual cilia analysed is indicated in the respective bar. Differences were highly significant by Student’s t -test, with P <0.01 (upper bar graph). The total level of ciliation is only mildly affected by Nek8 knockdown (lower bar graph; percentage of numeric counts of ciliated cells over total cells). ( f ) Fluorescence immunohistochemistry on kidney sections of wild-type (upper panels) and Nek8 −/− mice (lower panels), employing antibodies against ANKS6 (green) and acetylated tubulin (red). Positive ANKS6 signals at the ciliary base can only be identified in the wild type, not in Nek8 −/− cilia (scale bar, 5 μm). ( g , h ) Coexpression of myc-tagged ANKS6 truncation variants and FLAG-tagged wild-type NEK8 demonstrates the importance of the ANK-repeat domain for NEK8 binding and consecutive ciliary targeting of ANKS6 (scale bar, 2 μm; upper bar graph, percentage of numeric counts of ANKS6-positive cilia over total cilia; lower bar graph, percentual level of ciliation; the number of cells counted is indicated in each bar). Full size image Given the model in which NEK8 and ANKS6 form a distinct high-affinity subcomplex within the IC, we tested the hypothesis that NEK8 is required for ANKS6 localization to the IC. To this end, we analysed the subcellular localization of ANKS6 by immunofluorescence (IF) in IMCD cells harbouring a lentiviral Nek8 -specific short hairpin RNA construct. Although knockdown of endogenous Nek8 was incomplete, as determined by a residual ciliary IF signal with an antibody to endogenous NEK8, we found a significant reduction in ciliary ANKS6 staining ( Fig. 3d,e , upper chart). The level of ciliation was only mildly reduced in the Nek8 knockdown cells ( Fig. 3e , lower chart). We also performed fluorescent immunohistochemistry on kidney sections of wild type and Nek8 −/− mice. Although endogenous ANKS6 protein localized to the basal region of renal tubular epithelial cilia in wild-type kidneys, there was no detectable signal in the cilia of Nek8 −/− mice ( Fig. 3f and Supplementary Fig. 3 ), confirming the dependence of ANKS6 on NEK8 for ciliary IC localization. We also expressed FLAG-tagged NEK8 in mIMCD3 cells, along with the same myc-tagged ANKS6 truncations used in the above co-IPs. Consistent with the interaction pattern observed by co-IP, proper targeting of ANKS6 to the IC was exclusively dependent on the ANK-repeat domain, with partial ANK-domain truncations exhibiting reduced levels of ciliary localization ( Fig. 3g,h ). All these data support a model by which the NEK8 activator ANKS6 is targeted to the IC primarily through its interaction with NEK8. Recessive mutations in Anks6/Nek8 cause laterality defects From an N -ethyl- N -nitrosourea mouse mutagenesis screen for recessive mutations causing congenital heart defects (CHD), we recovered two independent mutants, ‘ Streaker ’ (MGI:5463579) and ‘ Roc ’ (MGI:5317588), exhibiting a spectrum of complex CHD associated with left–right asymmetry randomization. As the mutagenesis was conducted in the inbred C57BL6/J mouse strain, mutations in Streaker and Roc were readily recovered using whole mouse exome sequencing. As this was designed as a recessive screen, all of the homozygous mutations were considered as possible candidates, with genotyping analysis used to identify the pathogenic mutation as one consistently homozygous in all of the mutants. In this manner, Streaker was identified as having a pathogenic Anks6 missense substitution of the highly conserved methionine-187 to lysine within the ANK-repeat domain. In Roc , the pathogenic mutation was shown to be a missense substitution of the highly conserved isoleucine-124 to threonine in the kinase domain of NEK8. The latter represents the very first pathogenic Nek8 kinase domain mutation ( Supplementary Fig. 4a,b ). Both mutations were further validated by extensive breeding of the Roc and Streaker mutant lines, which has shown the consistent segregation of the mutant phenotypes with the respective Nek8 Roc and Anks6 Strkr mutations through multiple generations. Phenotypes of Anks6 Strkr and Nek8 Roc mutants were carefully analysed using a combination of necropsy examination to determine visceral organ situs and histopathology for the detailed diagnosis of CHD using episcopic confocal microscopy (ECM) [19] . The normal left–right pattern of visceral organ situs is referred to as situs solitus (SS). In the thoracic cavity, this is characterized by three lung lobes on the right and two on the left (as seen by necropsy view, although postcaval lobe anatomically connects to the right bronchial tree), a left-sided aortic arch and the heart apex pointing to the left (levocardia) ( Fig. 4a ). In the abdomen, stomach, spleen and pancreas are on the left ( Fig. 4a ). With defects in left–right patterning, there can be mirror symmetric reversal of visceral organ situs , referred to as situs inversus totalis ( Fig. 4b,j ), or randomization or discordant visceral organ situs as in heterotaxy ( Fig. 4c,k ). Heterotaxy was observed in approximately half of all Streaker and Roc mutants, with the remaining half equally divided between those with situs inversus totalis and SS ( Table 1 and Supplementary Tables 2 and 3 ). 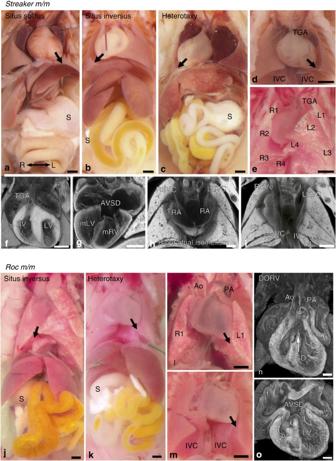Figure 4: HomozygousAnks6StrkrandNek8Rocmutants exhibit a ciliopathy syndrome. (a–i) HomozygousAnks6Strkrmutants exhibit a spectrum of left–right patterning defects and complex CHD. (a) SS, (b)situs inversusand (c)situs ambiguusor heterotaxy presentations in homozygousAnks6Strkrmutant mice. Note the presence of dextrocardia with the right-sided stomach in the heterotaxy mutant. (d) In a heterotaxy mutant, the aorta is transposed anterior to the pulmonary artery, yielding TGA. In addition, note the duplication of the inferior vena cava (IVC). (e) Heterotaxy mutants typically exhibit right pulmonary isomerism with four lung lobes bilaterally. (f–i) Histology and 3D reconstruction using ECM allowed detailed interrogation of intracardiac anatomy for CHD diagnosis. Shown areAnks6Strkrmutants exhibiting TGA with the aorta inserted into the RV (f); atrioventricular septal defects (AVSD) (g); right atrial isomerism with symmetrical insertion of the superior vena cava (RSVC and LSVC inh) into the left and right atria, respectively, and abnormal duplication of the IVC (i), and right pulmonary isomerism with four lung lobes bilaterally (i). (j–o) HomozygousNek8Rocmutants exhibit a spectrum of left–right patterning defects includingsitus inversus(j) and heterotaxy (k). (l) A mutant is shown exhibiting thoracicsituswith left pulmonary isomerism, as indicated by only one right and left lung lobe. (m) Duplicated IVC can also be observed. (n,o) Histological analysis with ECM showed double outflow right ventricle with positioning of both the aorta (Ao) and pulmonary artery (PA) over the RV (n) and a large ventricular septal defect (VSD). Also observed is an AVSD (o). Scale bars, 200 μm (black); 500 μm (white). Figure 4: Homozygous Anks6 Strkr and Nek8 Roc mutants exhibit a ciliopathy syndrome. ( a – i ) Homozygous Anks6 Strkr mutants exhibit a spectrum of left–right patterning defects and complex CHD. ( a ) SS, ( b ) situs inversus and ( c ) situs ambiguus or heterotaxy presentations in homozygous Anks6 Strkr mutant mice. Note the presence of dextrocardia with the right-sided stomach in the heterotaxy mutant. ( d ) In a heterotaxy mutant, the aorta is transposed anterior to the pulmonary artery, yielding TGA. In addition, note the duplication of the inferior vena cava (IVC). ( e ) Heterotaxy mutants typically exhibit right pulmonary isomerism with four lung lobes bilaterally. ( f – i ) Histology and 3D reconstruction using ECM allowed detailed interrogation of intracardiac anatomy for CHD diagnosis. Shown are Anks6 Strkr mutants exhibiting TGA with the aorta inserted into the RV ( f ); atrioventricular septal defects (AVSD) ( g ); right atrial isomerism with symmetrical insertion of the superior vena cava (RSVC and LSVC in h ) into the left and right atria, respectively, and abnormal duplication of the IVC ( i ), and right pulmonary isomerism with four lung lobes bilaterally ( i ). ( j – o ) Homozygous Nek8 Roc mutants exhibit a spectrum of left–right patterning defects including situs inversus ( j ) and heterotaxy ( k ). ( l ) A mutant is shown exhibiting thoracic situs with left pulmonary isomerism, as indicated by only one right and left lung lobe. ( m ) Duplicated IVC can also be observed. ( n , o ) Histological analysis with ECM showed double outflow right ventricle with positioning of both the aorta (Ao) and pulmonary artery (PA) over the RV ( n ) and a large ventricular septal defect (VSD). Also observed is an AVSD ( o ). Scale bars, 200 μm (black); 500 μm (white). Full size image Table 1 Summary of situs phenotypes in Anks6 Strkr and Nek8 Roc mutants*. Full size table Interestingly, Roc and Streaker heterotaxy mutants showed some differences in the distribution of visceral organ situs . All five Roc heterotaxy mutants exhibited levocardia, compared with only 7 of 20 Streaker heterotaxy mutants. Among Streaker heterotaxy mutants there was predominance of right pulmonary isomerism (11/20 RPI, 2/20 left pulmonary isomerism (LPI)), whereas among five Roc heterotaxy mutants only one exhibited RPI and two had LPI ( Table 1 ). Although three of five Roc heterotaxy mutants exhibited bilateral symmetric liver lobation, this was never observed in Streaker mutants ( Supplementary Tables 2 and 3 ). Complex CHDs in Anks6 Strkr and Nek8 Roc Streaker mutants with heterotaxy invariably exhibited complex CHD and died perinatally, while those with SS or situs inversus totalis largely exhibited normal cardiovascular anatomy and long-term postnatal survival ( Fig. 4f–i and Supplementary Tables 2 and 3 ). The complex CHD in Streaker mutants almost entirely consist of transposition of the great arteries (TGAs). Most heterotaxy mutants exhibited TGA ( Fig. 4d,f and Supplementary Movie 1 ), with several exhibiting the Taussig-Bing sub-type, with double-outlet right ventricle (RV), where both great arteries inserted into the RV ( Supplementary Table 2 ). Most heterotaxy mutants also exhibited atrioventricular septal defect ( Fig. 4g and Supplementary Movie 1 ). Some mutants exhibited right atrial isomerism, in which the atria show symmetrical insertion of the right versus left superior vena cava ( Fig. 4h ). Moreover, muscular or perimembranous ventricular septal defects ( Supplementary Table 2 ) were observed. The positioning of the inferior vena cava, normally on the anatomic right, can be seen on the right or the left, or duplicated bilaterally ( Fig. 4d,i ). Although Streaker mutants with heterotaxy usually showed RPI with three or four lung lobes bilaterally ( Fig. 4e,i ), the epiarterial branching pattern of the bronchi was often discordant, exhibiting LPI ( Supplementary Table 2 ). The liver, spleen and stomach showed discordant abdominal left–right patterning in nearly half of the heterotaxy mutants ( Supplementary Table 2 ). In Roc mutants, those with SS or situs inversus were without CHD and postnatally viable, similar to Streaker mutants. In Roc heterotaxy mutants, TGA was never observed and double-outlet RV was the only complex CHD detected, in conjunction with atrioventricular septal defect ( Fig. 4n,o and Supplementary Movie 2 ). As in Streaker mutants, Roc mutants with heterotaxy can exhibit right atrial isomerism, muscular or perimembranous ventricular septal defect, dual inferior vena cava and discordant abdominal situs ( Fig. 4m,n and Supplementary Table 3 ). Cilia motility unaffected in Anks6 Strkr and Nek8 Roc mutants Given the role of motile cilia in asymmetry determination, we investigated ciliary motility in airway epithelia of the trachea. Using videomicroscopy, we observed normal respiratory cilia motility in both Anks6 Strkr and Nek8 Roc mutants, indistinguishable from wild-type littermate controls ( Supplementary Movies 3 and 4 ). Airway epithelial cilia serve as a proxy for nodal cilia in many studies, as mutations affecting motile cilia function usually also disrupt airway cilia motility. However, given the normal respiratory cilia motility in both mutants, in combination with the striking asymmetry phenotype, we further investigated cilia motility in the embryonic node. As anticipated by the normal tracheal ciliary motility, Anks6 Strkr and Nek8 Roc mutants both exhibited normal nodal ciliary motility ( Supplementary Movie 5 ). Kidney defects in Anks6 Strkr and Nek8 Roc mutants Anks6 Strkr and Nek8 Roc mutants were also found to have kidney defects. These are characterized by widespread glomerular cysts ( Fig. 5b,e,h,i,n,r ) and cystic dilatation of renal tubules ( Fig. 5c,f,p,t ), predominantly along the corticomedullary junction. Although glomerulocystic disease is already remarkable in newborn animals, tubular cysts are initially small but mature significantly over weeks. Homozygous Anks6 Strkr mice without CHD survive for a longer term and analysis of 9- to 10-month-old mutants revealed prominent large corticomedullary cysts, along with secondary changes of interstitial consolidation, inflammation and scattered focal lymphoplasmocytic infiltrates ( Fig. 5m–r ). By that age, the glomerular cysts have also increased in number and size, occupying most of the cortical parenchyma ( Fig. 5n ). On occasion, Nek8 Roc mutants revealed urinary collecting system malformations with hydroureter, hydronephrosis and duplex kidneys. In the specimen shown in Fig. 5c,f , there is severe congenital obstructive uropathy with secondary consolidation and regression of the parenchymal band. On IF analysis of kidney sections using acetylated tubulin antibody, tubular epithelial cilia appeared shorter and reduced in density in Anks6 Strkr and Nek8 Roc mutants, as compared with wild type, whereas cystic epithelia in adult Anks6 Strkr mutants had longer cilia ( Fig. 5j–l,s,t ). 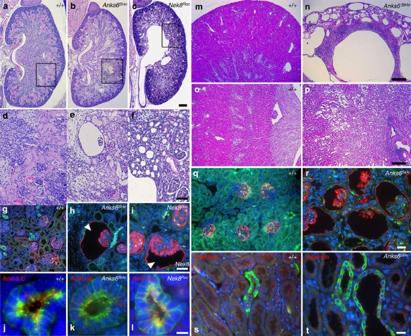Figure 5: Cystic kidney phenotypes inAnks6StrkrandNek8Rocmutants. (a–f) Haematoxylin and eosin-stained kidney sections of newborn wild-type (a,d), homozygousAnks6Strker(b,e) andNek8Rocmutant mice (c,f). In theAnks6mutant kidney, note the presence of widespread cystic tubular dilatation throughout the cortex and medulla, along with a number of markedly enlarged glomerular cysts. TheNek8Rocmutants showed hydronephrosis with hydroureter and cystic tubular dilatation throughout the parenchyma along with some small glomerular cysts (scale bar, 100 μm). (g–i) T1α (red, glomeruli),Dolichos biflorusagglutinin (DBA; green, collecting ducts) and DAPI (blue, nuclei) staining in these same kidneys showed cystic dilatation of Bowman’s space in the glomerulus in theAnks6(h) andNek8(i) mutants (scale bar, 10 μm). (j–l) Acetylated tubulin (red, cilia), DBA (green, collecting ducts) and DAPI (blue, nuclei) staining shows the presence of shortened cilia in the mutantAnks6StrkrandNek8Rocnewborn kidneys (scale bar, 10 μm). (m–p) Haematoxylin and eosin-stained kidney sections of adult wild-type (m,o) and homozygousAnks6Strkr(n,p) adult kidneys showed large glomerular cysts throughout the cortex and cystic tubular dilatation along the corticomedullary junction of the kidney, along with inflammatory mononuclear cell infiltrates in the mutant (n). Scale bar, 100 μm. (q,r) T1α (red, glomeruli), DBA (green, collecting ducts) and DAPI (blue, nuclei) staining of adult kidneys showed cystic dilatation of Bowman’s space in the glomerulus in theAnks6mutant (r; scale bar, 10 μm). (s,t) Acetylated tubulin (red, cilia), DBA (green, collecting ducts) and DAPI (blue, nuclei) staining of adult kidneys showed cystic dilatation of the collecting ducts and nephrons in theAnks6mutant (t). Note that tubular epithelia are ciliated in both control and mutant (scale bar, 5 μm). Figure 5: Cystic kidney phenotypes in Anks6 Strkr and Nek8 Roc mutants. ( a – f ) Haematoxylin and eosin-stained kidney sections of newborn wild-type ( a , d ), homozygous Anks6 Strker ( b , e ) and Nek8 Roc mutant mice ( c , f ). In the Anks6 mutant kidney, note the presence of widespread cystic tubular dilatation throughout the cortex and medulla, along with a number of markedly enlarged glomerular cysts. The Nek8 Roc mutants showed hydronephrosis with hydroureter and cystic tubular dilatation throughout the parenchyma along with some small glomerular cysts (scale bar, 100 μm). ( g – i ) T1α (red, glomeruli), Dolichos biflorus agglutinin (DBA; green, collecting ducts) and DAPI (blue, nuclei) staining in these same kidneys showed cystic dilatation of Bowman’s space in the glomerulus in the Anks6 ( h ) and Nek8 ( i ) mutants (scale bar, 10 μm). ( j – l ) Acetylated tubulin (red, cilia), DBA (green, collecting ducts) and DAPI (blue, nuclei) staining shows the presence of shortened cilia in the mutant Anks6 Strkr and Nek8 Roc newborn kidneys (scale bar, 10 μm). ( m – p ) Haematoxylin and eosin-stained kidney sections of adult wild-type ( m , o ) and homozygous Anks6 Strkr ( n , p ) adult kidneys showed large glomerular cysts throughout the cortex and cystic tubular dilatation along the corticomedullary junction of the kidney, along with inflammatory mononuclear cell infiltrates in the mutant ( n ). Scale bar, 100 μm. ( q , r ) T1α (red, glomeruli), DBA (green, collecting ducts) and DAPI (blue, nuclei) staining of adult kidneys showed cystic dilatation of Bowman’s space in the glomerulus in the Anks6 mutant ( r ; scale bar, 10 μm). ( s , t ) Acetylated tubulin (red, cilia), DBA (green, collecting ducts) and DAPI (blue, nuclei) staining of adult kidneys showed cystic dilatation of the collecting ducts and nephrons in the Anks6 mutant ( t ). Note that tubular epithelia are ciliated in both control and mutant (scale bar, 5 μm). Full size image NEK8 kinase activity is essential for ciliopathic phenotypes We sought to determine the mechanism of pathogenicity of the Anks6 Strkr and Nek8 Roc alleles. On investigation of the subcellular localization in mIMCD3 cells, we found that overexpressed ANKS6 M187K protein co-localized with FLAG-NEK8 to the IC, to a comparable level as wild-type ANKS6 ( Fig. 6a,b ). On immunohistochemistry of Anks6 Strkr kidney sections, we also identified the presence of ANKS6 protein in the base of tubular epithelial cilia ( Fig. 6c , middle, and Supplementary Fig. 5 ). However, on co-IP analysis we found a significantly reduced level of co-precipitating ANKS6 M187K compared with wild type, or the truncation variant that lacks the first ANK repeat ( Fig. 6d and Supplementary Fig. 4c ). The interaction between ANKS6 M187K and NEK8 was salt insensitive, as seen with wild-type ANKS6, but occurred at a much lower affinity ( Fig. 6e ). Given the low-affinity interaction, no phosphorylation activity was detected in the kinase assay ( Fig. 6f ). Although IF and immunohistochemistry reveal that mutant protein is still present in cilia, IP under stringent ionic strength is more sensitive to differences in binding affinity and reduced the NEK8 kinase activity. 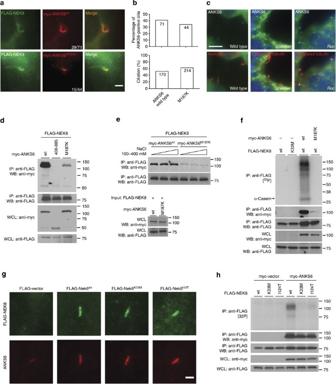Figure 6:Anks6M187KandNek8I124Tmutations exert their pathogenicity through a functional inactivation of the NEK8 kinase. (a,b) IF analysis of FLAG-tagged NEK8 with myc-tagged wild type and ANKS6M187Kmutant proteins suggests that mutant protein is capable of localizing to the IC (scale bar, 2 μm). (c) Fluorescence immunohistochemistry of kidney sections of wild type (left),Anks6Strkrmice (middle) andNek8Rocmice (right), employing antibodies against native ANKS6 protein (green) and acetylated tubulin (red; scale bar, 5 μm). ANKS6 positivity at the base of renal tubular epithelial cilia is noted in all examined genotypes. (d) Co-IP of myc-tagged wild-type ANKS6 (positive control), the ΔANK-repeat domain (negative control) and the ANKS6M187Kmutant with FLAG-Nek8 reveals a markedly reduced binding affinity of the mutant. (e) Co-IP of wild-type and mutant ANKS6 with NEK8 at different NaCl concentrations. The interaction of NEK8 with the ANKS6M187Kmutant occurs at a lower affinity than with the wild type, but is also independent of ionic strength. (f) Co-IP and kinase assays of NEK8 in the presence or absence of ANKS6 and the ANKS6M187Kmutation. The co-precipitated ANKS6M187Kmutant protein fails to sufficiently stimulate NEK8 phosphorylation activity. (g) All examined NEK8 alleles (wild type, K33M and I124T) are capable of translocating to the IC and to recruit ANKS6, as shown by IF of FLAG-NEK8-transfected IMCD shNek8 cells (anti-FLAG, green), and counterstain for endogenous ANKS6 (red; scale bar, 2 μm). (h) Co-IP and kinase assays reveal that NEK8I124Tinteraction with ANKS6 is unimpaired, as compared with the wild type. However, the NEK8I124T/ANKS6 complex is functionally ‘kinase dead’ and reveals a negligible extent of phosphorylation activity, as compared with ANKS6-associated wild-type NEK8 (positive control) and NEK8K33M(negative control). Figure 6: Anks6 M187K and Nek8 I124T mutations exert their pathogenicity through a functional inactivation of the NEK8 kinase. ( a , b ) IF analysis of FLAG-tagged NEK8 with myc-tagged wild type and ANKS6 M187K mutant proteins suggests that mutant protein is capable of localizing to the IC (scale bar, 2 μm). ( c ) Fluorescence immunohistochemistry of kidney sections of wild type (left), Anks6 Strkr mice (middle) and Nek8 Roc mice (right), employing antibodies against native ANKS6 protein (green) and acetylated tubulin (red; scale bar, 5 μm). ANKS6 positivity at the base of renal tubular epithelial cilia is noted in all examined genotypes. ( d ) Co-IP of myc-tagged wild-type ANKS6 (positive control), the ΔANK-repeat domain (negative control) and the ANKS6 M187K mutant with FLAG-Nek8 reveals a markedly reduced binding affinity of the mutant. ( e ) Co-IP of wild-type and mutant ANKS6 with NEK8 at different NaCl concentrations. The interaction of NEK8 with the ANKS6 M187K mutant occurs at a lower affinity than with the wild type, but is also independent of ionic strength. ( f ) Co-IP and kinase assays of NEK8 in the presence or absence of ANKS6 and the ANKS6 M187K mutation. The co-precipitated ANKS6 M187K mutant protein fails to sufficiently stimulate NEK8 phosphorylation activity. ( g ) All examined NEK8 alleles (wild type, K33M and I124T) are capable of translocating to the IC and to recruit ANKS6, as shown by IF of FLAG-NEK8-transfected IMCD shNek8 cells (anti-FLAG, green), and counterstain for endogenous ANKS6 (red; scale bar, 2 μm). ( h ) Co-IP and kinase assays reveal that NEK8 I124T interaction with ANKS6 is unimpaired, as compared with the wild type. However, the NEK8 I124T /ANKS6 complex is functionally ‘kinase dead’ and reveals a negligible extent of phosphorylation activity, as compared with ANKS6-associated wild-type NEK8 (positive control) and NEK8 K33M (negative control). Full size image Subsequently, we investigated consequences of the Nek8 Roc allele regarding subcellular localization, ANKS6 recruitment and phosphorylation activity. NEK8 I124T is capable of localizing to the IC, as well as the wild type or the engineered ‘kinase-dead’ NEK8 K33M protein. Transfections and IF were performed in mIMCD3 shNek8 cells and all three transfected Nek8 alleles rescued IC localization of endogenous ANKS6, revealed by anti-ANKS6 counterstaining ( Fig. 6g ). On immunohistochemistry of Roc kidney sections, we also found ANKS6 labelling at the base of renal tubular epithelial cilia ( Fig. 6c , right, and Supplementary Fig. 5 ). On co-IP, ANKS6 binding to NEK8 I124T was unimpaired and the levels of co-precipitating ANKS6 protein were comparable between NEK8 wild type, NEK8 K33M and NEK8 I124T ( Fig. 6h , lower panels). However, in the kinase assay NEK8 I124T appeared functionally ‘kinase-dead’, exhibiting dramatically reduced activity in the presence of ANKS6 ( Fig. 6h , upper panel, and Supplementary Fig. 4d ). We conclude that selective disruption of NEK8 kinase activity is responsible for the severe phenotype that is comparable to that found in the targeted Nek8 deletion. Together, these results provide evidence of an essential role for the kinase activity of NEK8 in the regulation of left–right patterning and renal morphogenesis. We note the phenotypes in Roc and Streaker mutants arise from single amino acid substitutions that each perturb NEK8 kinase function, either through the direct disruption of phosphorylation activity or through impaired interaction with its activator. Despite the characterization of numerous human and rodent mutations of IC proteins, the function of this ciliary subdomain remains poorly understood. Our study shows that ANKS6, a known interaction partner of the IC kinase NEK8 (as previously reported [18] ), has unique properties as an NEK8 kinase activator and phosphorylation substrate. We show the NEK8/ANKS6 interaction as structurally and functionally distinct within the IC interaction network, and required for proper targeting of ANKS6 to the IC. Two novel autosomal-recessive missense mutations in mouse Anks6 and Nek8 demonstrate for the first time the specific importance of NEK8 kinase activity in developmental signalling. Noteworthy is the fact that the Streaker mutation in Anks6 (M187K) and the Roc mutation in Nek8 (I124T) give rise to very similar phenotypes of left–right asymmetry randomization, CHD and cystic kidneys. Most importantly, these missense mutations, both causing deactivation of NEK8 kinase function, are sufficient to phenocopy the full spectrum of syndromic phenotypes seen in mutants with the NEK8 targeted deletion, as well as mutants with null mutations in other IC genes. Together, our data highlight the importance of NEK8 kinase function and its activator, ANKS6, in early embryonic patterning of the left–right body axis and in cardiovascular and renal morphogenesis. Choi et al . [17] hypothesized that renal cystogenesis occurs through NEK8 kinase activities related to DNA replication stress, based on their observation that the human NEK8 G442V mutation (orthologous to the murine jck allele) rendered the NEK8 kinase inactive. Our results highlight a different aspect of NEK8 kinase function. We do not observe a striking difference in kinase activity in the setting of the murine Nek8 jck allele; however, we observe a requirement for ANKS6 in stimulating kinase activity. The mechanistic explanation for a putative kinase activity reducing effect of an RCC1 domain (non-kinase domain) mutation remains elusive. It is noted that the jck mouse exhibits no laterality defects, in contrast to the Nek8 -targeted deletion and the Nek8 Roc mutant. Consequently, we propose a developmental signalling pathway specific to the IC, which is contingent on NEK8 kinase activity, and which sufficiently explains situs determination and cystic kidney phenotypes. In a study by Hoff et al . [18] , ANKS6 was first identified as an IC component and NEK8 interaction partner. Hoff et al . [18] postulated that ANKS6 organizes the assembly of a ciliary NEK8-INVS-NPHP3 module, maintains connections to a set of mitochondrial proteins and is subject to regulation by HIF1AN and the hypoxia pathway. Discordant with Hoff et al . [18] , we demonstrate that ANKS6 is downstream of NEK8 in the IC assembly hierarchy and exhibits a uniquely strong and functional interaction with NEK8, which is necessary for a NEK8-mediated phosphorylation pathway. Our study leads to questions regarding whether ANKS6 represents the only physiological NEK8 substrate, or whether there are additional NEK8/ANKS6-kinase-dependent or -independent signalling outputs of the IC. Sohara et al . [20] presented indirect evidence for NEK8-dependent phosphorylation of polycystin-2, but we were unable to detect any radioactive phosphate incorporation using immunoprecipitated polycystin-2 as a substrate in our in vitro assay (unpublished data). Similarly, ANKS3, a different member of the family of ANK- and SAM-domain-containing proteins that we identified as an NEK8 interaction partner ( Fig. 1b ), is not a substrate of NEK8-mediated phosphorylation (unpublished data). Notably, although the ANK-repeat domain of ANKS6 appears sufficient to stimulate NEK8 kinase activity, ciliopathic ANKS6 mutations are also found in the SAM domain. This is true for the rat Han:SPRD cy/+ model of polycystic kidney disease [21] and for at least one highly pathologic human ANKS6 mutation (A649:21) [18] . We show that SAM-domain truncations do not affect the general activation mechanism of NEK8-dependent phosphorylation. Thus, ciliopathic mechanisms of ANKS6 SAM-domain mutations are not necessarily the same as those of reduced NEK8 kinase activity. Further studies will be required to distinguish SAM-domain functions from the NEK8 activator functions of ANKS6. The phenotypic spectrum of left–right asymmetry randomization, CHD and cystic kidney malformations represents a characteristic syndrome of perturbed IC-mediated signalling, exemplified here by the Roc and Streaker mutant mice, and consistent with findings in the inv/inv mouse and the NPHP3 and Nek8 knockout mouse models [5] , [6] , [7] . It is phenotypically distinct from other ciliopathy syndromes, including the Joubert-syndrome-related disorders, Meckel–Gruber syndrome or Bardet–Biedl syndrome, and the lack of reported neural tube closure and CNS patterning defects, retinitis pigmentosa or obesity suggests that the IC regulates a different and very specific set of ciliary functions. We note IC disruption having not been directly implicated in motile ciliary dysfunction. Notably, previous work in the inv/inv mouse demonstrated normal nodal ciliary motility but a defective nodal flow pattern [22] . At that time, an abnormally shaped node was hypothesized as the origin of the defective flow and heterotaxy, but more recently proposed models may justify revisiting nodal flow and signalling in the inv/inv mouse [23] , [24] , [25] . Models of situs determination propose that the nodal flow generated by monocilia in the floor of the ventral node deflects non-motile cilia of the perinodal crown cells situated at the crest of the node [25] . This mechanical deflection is proposed to generate a calcium transient on the left side of the node that is required for left-sided expression of asymmetry genes, such as Nodal [23] , [24] , [25] . It has been proposed that polycystin-2 and polycystin-1-like-1 may play a key role in this mechanosensory transduction. Based on our findings, we propose an attractive unifying hypothesis that NEK8/ANKS6-mediated signalling in the primary cilia of perinodal crown cells may regulate polycystin function required for left–right patterning and thus provide a mechanistic link between the IC, and phenotypic outcomes of situs determination and polycystic kidneys in the Anks6 Strkr and Nek8 Roc mutants. Vectors and complementary DNA clones We used standard PCR and cloning techniques to generate rat Anks6 , mouse Nek8 and human INVS and NPHP3 expression constructs, and the respective missense and truncation mutants. Expression plasmids were based on a modified pcDNA3.1(+) vector (Life Technologies), to include N-terminal 3XFLAG-, myc-, LAP- or V5-tags. PCR templates of rat Anks6 were generously provided by Dr Elizabeth Bryda, University of Missouri [26] . PCR primer sequences are published in Supplementary Table 4 . Antibodies The following antibodies were used for western blotting (WB) and IF: anti-FLAG M2, anti-FLAG rabbit polyclonal (1:5,000 WB and IF, Sigma-Aldrich), anti-c-Myc 9E10, anti-c-Myc rabbit polyclonal (1:5,000 WB and IF, Sigma-Aldrich), anti-acetylated tubulin 6-11B-1 (1:20,000 IF on cell culture cells, 1:5,000 IF on kidney sections, Sigma-Aldrich), anti-ANKS6 (1:1,000; Sigma-Aldrich), anti-V5 Pk1 (1:5,000, Serotec) and anti-NEK8 (1:1,000 (ref. 10 )). Secondary antibodies used in WB were goat-anti-mouse-horseradish peroxidase and goat-anti-rabbit-horseradish peroxidase (1:10,000, Jackson ImmunoResearch). Secondary antibodies used in cultured cell IF were the AlexaFluor 488 goat anti-rabbit IgG and AlexaFluor 594 goat anti-mouse IgG (1:1,000, Life Technologies). For kidney sections, we used AlexaFluor 568 F(ab′) 2 fragment of goat anti-mouse IgG for anti-acetylated tubulin 6-11B-1 and AlexaFluor 568 goat anti-hamster IgG for T1α (1:1,000, Life Technologies). Cell culture and transfection HEK 293T/17, mIMCD3 and LLC-PK1 cells (ATCC; CRL-11268, CRL-2123 and CL-101, respectively) were cultured in DMEM containing 10% fetal bovine serum at 37 °C and 5% CO 2 . Transfection of HEK 293T/17 cells for IP and kinase reactions was carried out in 10-cm dishes using Polyfect (QIAGEN), according to the manufacturer’s protocol. LLC-PK1 and mIMCD3 cells were transfected for IF using Lipofectamine LTX (Life Technologies) in 12-well plates, according to the manufacturer’s manual. Retroviral transduction of mIMCD3 cells with a FLAG- Nek8 transgene was described previously [27] . Briefly, the pcDNA3.1(+) 3XFLAG- Nek8 construct described above was cut with NheI, the site was blunted with T4 DNA polymerase and the insert was excised by a second cut with XhoI. The fragment was ligated into pBABE-Neo (Addgene; 1765) and digested with NaeI/SalI. The 3XFLAG- Nek8 pBABE-Neo vector was co-transfected into 293T cells with pCMV-VSV-G (Addgene; 8454) and pUMVC (Addgene; 8449). Cell culture supernatant was removed 2 days after transfection, filtered through a 0.45-μm syringe filter and applied on 50% confluently growing mIMCD3 cells. After another 2 days of culture, media were changed and selection with Neomycin was conducted for 2 weeks, resulting in a polyclonal 3XFLAG- Nek8 -expressing mIMCD3 cell line. Cell lysis and Immunoprecipitation Sixteen hours after transfection, HEK 293T/17 cells were washed in PBS and lysed in HBST400/0.2 (HEPES-NaOH 25 mM, pH 7.5, NaCl 400 mM, 0.2% Triton X-100) for NEK8/ANKS6 co-IP experiments and HBST100/1.0 (NaCl 100 mM, 1.0% Triton X-100) for all other preparations, unless otherwise indicated. Whole Cell Lysate (WCL) samples for SDS–PAGE were brought to 1 μg μl −1 with water and 4 × SDS–PAGE sample buffer. For IP, typically 1.5 mg of protein sample was incubated with 15 μl bed volume of anti-FLAG-M2 affinity gel (Sigma-Aldrich) in a volume of 1 ml for 1 h at 4 °C. Immune complexes were washed four times and eluted into SDS–PAGE sample buffer. For proteomics, we employed total protein of three 225 cm 2 flasks of confluently growing, serum-starved wild-type mIMCD3 cells (control) and mIMCD3 cells stably transduced with FLAG- Nek8 . We used HBST100/1.0 for lysis and IP, and an additional ultracentrifugation step at 100,000 g was performed before addition of affinity resin. For silver staining, we used the Novex SilverQuest kit (Life Technologies), according to the manufacturer’s protocol. Alternatively, IP complexes were eluted with 3 × FLAG peptide and submitted for mass spectrometric analysis without prior PAGE. Proteomic analysis was carried out at the Taplin Mass Spectrometry facility (Harvard Medical School). The experiments in Fig. 1a,b were each carried out once. SDS–PAGE and WB SDS–PAGE was performed on Mini PROTEAN gels (Bio-Rad) in a Tris/Glycine/0.1% SDS buffer system. Gels were blotted on Nitrocellulose (Protran BA 83, Whatman) in Tris/Glycine/0.1% SDS/20% methanol. Blots were blocked in 2.5% BSA/TBST, primary antibody solutions were in 1% BSA/TBST, secondary antibodies were in TBST. Final detection was carried out with the Western Lightning ECL Pro reagent (Perkin Elmer). Individual results from western blottings were repeated multiple times. Uncropped scans of western blottings from the main figures are included into the Supplementary Information section ( Supplementary Fig. 6 ). In vitro kinase assays FLAG-tagged NEK8 immunocomplexes were resuspended in 30 μl kinase buffer (25 mM HEPES-NaOH, pH 7.5, 100 mM NaCl, 0.2% Triton X-100, 5 mM β-glycerophosphate, 5 mM MnCl 2 , 2 mM dithiothreitol, 6.7 mM final concentration non-radioactive ATP and 2 μCi/assay γ[ 32 P]-ATP (Perkin Elmer). Assays were incubated at 30 °C for 30 min and quenched by addition of 10 μl 4 × SDS–PAGE sample buffer. After SDS–PAGE, gels were fixated in 10% v/v acetic acid, 40% v/v ethanol and 5% v/v glycerol in ultrapure water, before heated vacuum drying and exposure of autoradiography films. IF microscopy Transfected and serum-starved LLC-PK1 and mIMCD3 cells were washed and fixed in 3.7% formaldehyde in MTSB (50 mM PIPES-KOH, pH 7.0, 5 mM EGTA, 5 mM MgSO 4 , 25 mM KCl), permeabilized in MTSB/0.4% Triton X-100 and blocked in 2% BSA in MTSB/0.1% Triton X-100. Primary and secondary antibodies were applied for 1 h each in the same blocking solution. Coverslips were incubated in DAPI (4',6-diamidino-2-phenylindole) and mounted in Vectashield (Vector Labs). The slides were mounted on the stage of a Nikon Eclipse Ti inverted microscope equipped with a Nikon Plan Apo Fluor 60xA 1.4 NA objective lens and a CoolSnap-HQ (Photometrics). IF images and statistical data ( Figs 3d,e,g,h and 6a,b ) were derived from single large-scale transfections each, assessing sample sizes between 669 and 2041 cells from at least 40 individual high-power fields. No statistical method was used to predetermine sample sizes. The estimate of variation is reflected by s.d. in graphs ( Fig. 3e ). Acquisition settings were kept constant for all samples so that valid comparisons could be made between measurements from different data sets. Acquisition parameters were set within the linear range of the charge-coupled device camera detection. Fluorescence histochemistry and immunohistochemistry Seven-micrometre kidney paraffin sections were cut and transferred to slides (Superfrost plus, Fisher Scientific). Sections were dewaxed (Safeclear, Fisher Scientific) and rehydrated with graded aqueous isopropanol. Antigen retrieval was carried out with 10 mM sodium citrate, pH 6, in an autoclave (250 °F for 40 min). Sections were blocked for 30 min (4% non-immune goat serum, 0.1% cold water fish skin gelatin, 0.1% Triton X-100, 0.1% Tween-20 in TBS). One per cent BSA and 0.05% SDS were added to the blocking solution in the ANKS6-labelling experiments to reduce background. Incubation with primary antibodies/lectin was carried out overnight at 4 °C: T1α (1:1,000, Developmental Studies Hybridoma Bank, University of Iowa), fluorescein-conjugated Dolichos biflorus agglutinin (1:200, Vector Labs), anti-acetylated tubulin, anti-ANKS6 and secondary antibodies as above. For anti-ANKS6 IF, a biotin layer was employed to enhance labelling of ANKS6, requiring endogenous biotin to be blocked (Avidin/Biotin blocking kit, Life Technologies) before application of the biotin-conjugated secondary antibody (Fab fragment of goat anti-rabbit IgG at 1:250, Jackson Immunochemicals) and streptavidin-Alexa 488 at 1:400. Slides were incubated in DAPI and mounted with Prolong Gold (Life Technologies). Imaging was carried out using a Zeiss Axiovert 200 microscope and OpenLab 3.1.5 software (Improvision). Mouse mutagenesis screen and phenotyping analysis Studies involving the Streaker and Roc mutant mice were approved by the Institutional Animal Care and Use Committee of the University of Pittsburgh and conform to NIH guidelines. C57BL6/J mice were chemically mutagenized and subject to a two-generation backcross breeding scheme for recovery of recessive mutations causing CHDs as previously described [28] . The phenotyping screen was conducted using non-invasive fetal echocardiography [29] and the mutants recovered were further analysed by necropsy followed by two-dimensional (2D) and three-dimensional (3D) reconstructions using ECM of the paraffin-embedded specimen [19] . The necropsy analysis allowed the determination of most visceral organ situs phenotypes, including duplex kidneys and moderate-to-severe kidney cysts. Briefly, ECM imaging entails capturing fluorescence images of the paraffin block face serially, as it is being sectioned on a Leica SM2500 microtome using an Large Scale Imaging (LSI) confocal macroscope, to generate registered 2D image stacks. The 2D image stacks were digitally resectioned or 3D volume rendered using Osirix software. The ECM 2D image stacks observed in different imaging planes and 3D reconstructions allowed full assessment of intracardiac anatomy to arrive at a complete and systematic diagnosis of complex CHD. Using the ECM 2D imaging stacks, we were also able to determine the precise left–right bronchial branching and lung lobation pattern. Kidneys were further processed for standard histology (haematoxylin/eosin) and IF. Animal experiments were not randomized and the investigators were not blinded to allocation during experiments and outcome assessment. Whole mouse exome-sequencing analysis and mutation recovery Genomic DNA from one Streaker and one Roc mutant were processed for whole exome capture using the Agilent SureSelect Mouse All Exon array (50 Mb), followed by pair-end sequencing using the Illumina HiSeq 2000. Reads were mapped to C57BL6 reference genome (mm9) and analysed using CLCBio Genomic Workbench software. An average 50 × coverage was obtained for each exome, and variants were annotated using annovar and filtered using custom scripts. For the Streaker mutant, 11 homozygous coding mutations were recovered from the exome-sequencing analysis. Subsequent genotyping analysis identified the Anks6 M187K mutation as the only mutation consistently homozygous across all mutants recovered in this line, thus indicating it is the disease-causing pathogenic mutation. Similarly, for the Roc mutant line, ten homozygous coding mutations were identified, with Nek8 I124T identified as the pathogenic mutation that is consistently homozygous in all of the mutants. Further breeding of both lines through multiple generations have validated the Anks6 M187K and Nek8 I124T mutations as the pathogenic mutations in the Streaker and Roc mutant lines, respectively. Tracheal and embryonic node cilia videomicroscopy Tracheae were dissected and prepared for videomicroscopy as previously described [30] . Briefly, this entailed placing the tracheal luminal side down on to a 35-mm glass-bottomed culture dish (Willco Wells B.V, Netherlands), placing a 0.3-mm-thick silicone sheet (AAA Acme Rubber Co., AZ) with a small window cut out over the trachea and then placing a round glass coverslip (FisherBrand, USA) on top to secure it on the 35-mm dish. To record the motile cilia of the embryonic node, E7.75 embryos were collected in L15 medium and the node was dissected from the embryo proper and placed onto a glass slide in which a small chamber was constructed, using 0.3-mm-thick silicone sheet. The chamber was filled with L15 medium and covered with a glass coverslip to allow imaging of cilia motility, using a Leica DMIRE2 inverted microscope equipped with a × 100 oil objective and Differential Interference Contrast (DIC) optics. High Speed movies (200 fps) were collected using a Phantom v4.2 camera (Vision Research, NJ) and saved in the AVI format. How to cite this article: Czarnecki, P. G. et al . ANKS6 is the critical activator of NEK8 kinase in embryonic situs determination and organ patterning. Nat. Commun. 6:6023 doi: 10.1038/ncomms7023 (2015).